Whole Genome Association Study of the Plasma Metabolome Identifies Metabolites Linked to Cardiometabolic Disease in Black Individuals Integrating genetic information with metabolomics has provided new insights into genes affecting human metabolism. However, gene-metabolite integration has been primarily studied in individuals of European Ancestry, limiting the opportunity to leverage genomic diversity for discovery. In addition, these analyses have principally involved known metabolites, with the majority of the profiled peaks left unannotated. Here, we perform a whole genome association study of 2,291 metabolite peaks (known and unknown features) in 2,466 Black individuals from the Jackson Heart Study. We identify 519 locus-metabolite associations for 427 metabolite peaks and validate our findings in two multi-ethnic cohorts. A significant proportion of these associations are in ancestry specific alleles including findings in APOE, TTR and CD36 . We leverage tandem mass spectrometry to annotate unknown metabolites, providing new insight into hereditary diseases including transthyretin amyloidosis and sickle cell disease. Our integrative omics approach leverages genomic diversity to provide novel insights into diverse cardiometabolic diseases. Disturbed metabolism plays a central role across a spectrum of pathological processes from cancer to cardiometabolic disease [1] , [2] . Metabolomics aims to systematically measure small molecules and provides a snapshot of metabolic activity, capturing both genetic and environmental influences on disease pathogenesis [3] . The integration of genomics and metabolomics has been increasingly leveraged in efforts to identify bioactive metabolites linked to human disease, as large-scale genome-wide association studies (GWAS) have played a critical role in our understanding of loci that affect disease risk. Previous GWAS of the metabolome has identified associations between hundreds of genomic loci across a broad range of metabolite classes, including amino acids, nucleosides, and lipids among others [4] , [5] , [6] , [7] , [8] , [9] , [10] , [11] , [12] , [13] , [14] , [15] , [16] , [17] , [18] , [19] , [20] , [21] , [22] , [23] , [24] . While prior studies have ranged in sample sizes from several hundred to a few thousand individuals, a recent study performed a GWAS meta-analysis across several large cohorts for 171 metabolites (in up to 86,507 individuals) measured using various metabolomic profiling platforms, including liquid chromatography-mass spectrometry (LC-MS) and nuclear magnetic resonance (NMR) spectroscopy [23] . This cross-platform analysis highlighted the robustness of findings in metabolomics GWAS and the ability to detect clinically relevant associations, helping to illuminate biology in both common diseases such as diabetes and rare conditions such as macular telangiectasia type II. Despite these efforts, the vast majority of metabolomics GWAS to date have been undertaken in cohorts of European ancestry, limiting the opportunity to leverage genomic diversity for biological discovery [25] , [26] , [27] . Individuals of African ancestry are more genetically diverse than those of European ancestry [28] , and carry ancestry-specific mutations which may illuminate biology and therapeutic strategies in cardiometabolic disease [29] . Further, most GWAS of the metabolome to date have used genotyping arrays with measurement of a limited set of tag single nucleotide polymorphisms (SNP) with the imputation of remaining variants, limiting the ability to accurately assess low-frequency protein-coding and non-coding variation. Finally, while tools for unbiased metabolomic profiling can now measure hundreds of known metabolites as well as thousands of unknown metabolite peaks [30] , [31] , the latter have eluded definitive compound identification, thus limiting biological insight into locus-metabolite associations. There are significant challenges in unknown metabolomic profiling, and attempts at further annotating these peaks in prior GWAS have been limited. First, unknown metabolite peaks must be separated from background noise and adduct ions of known and other unknown metabolites [32] . In addition, chemical identification of unique peaks requires downstream resource-intensive processes for structural elucidation, identification including the acquisition of product ion mass spectra (MS/MS) to generate metabolite fragmentation data as “chemical fingerprints” that can help improve compound identification [33] . We have previously demonstrated proof-of-principle suggesting the utility of integrating LC-MS of unknown peaks with genetic findings. For example, when peak levels map to solute carriers or enzymes with known functions, including substrates and products, this may help narrow the potential compound matches for chemical standard validation [34] . However, this has remained an arduous process, limiting its application in metabolomics GWAS of unknown peaks in large population-based studies. To extend prior work, we performed a genome-wide association study integrating whole genome sequencing (WGS) of 2,291 metabolite peaks in 2466 participants from the Jackson Heart Study (JHS), a Black epidemiological cohort in Jackson, Mississippi, and validated findings in the Multi-Ethnic Study of Atherosclerosis (MESA; n = 995) and Health, Risk Factors, Exercise Training and Genetics Family Study (HERITAGE; n = 658). Beyond confirming prior known locus-metabolite associations in a Black cohort—an important next step to test the generalizability of prior work—we highlight many novel findings, including associations in ancestry-specific alleles for heritable conditions more commonly observed in Black individuals, including transthyretin amyloidosis and sickle cell disease. We acquired MS/MS on metabolite features and have integrated WGS findings and recently developed bioinformatic tools that leverage MS fragmentation data for more efficient annotation and identification of unknown metabolite peaks. We have developed and made available an extensive sample library of metabolite peaks, linking MS/MS spectra, genomic associations, and clinical traits that can be leveraged for annotation and identification of unknown metabolites implicated in diverse disease processes. Our integrative omics approach highlights the value of whole genome sequencing analysis of the metabolome in diverse populations for biological discovery and contributes to a roadmap for the identification of metabolites implicated in human disease. We performed a whole genome association study (WGAS) in 2466 Black participants from JHS on 30,672,656 variants limited to an allele count of at least five against 2291 metabolites (337 known metabolites and 1954 unknown metabolites peaks; Fig. 1 ). 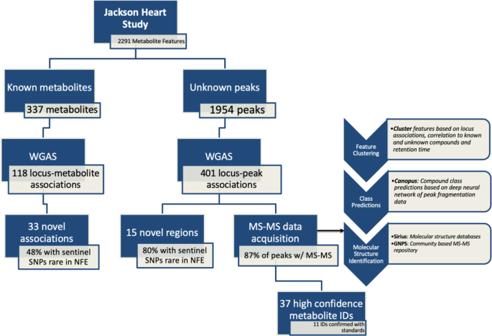Fig. 1: Whole Genome Association Study of known and unknown metabolites in the Jackson Heart Study. Flow diagram detailing whole genome association study of the metabolome, main results, and subsequent bioinformatic pipeline for unknown metabolite identification. Rare minor allele frequency is defined as <1% in NFE using gnomAD. Confirmation of metabolite identities was limited to commercially available metabolite standards. WGAS whole genome association study, MS mass spectrometry; NFE non-Finish Europeans, GNPS global natural product social networking. Clinical characteristics of the study population are detailed in Supplementary Table 1 . At a Bonferroni threshold of significance of 8E-11 (based on 5E-8 /602 principal components, which explain 95% of the variance in metabolite peak levels), there were 519 locus-metabolite associations, representing 427 metabolite peaks and 226 sentinel SNPs (Fig. 2 ). Of these, 118 locus-metabolite associations were determined from known metabolite analysis, representing 91 distinct metabolites. Comparison to prior GWAS of plasma metabolites, using publicly available summary statistics through PhenoScanner V2 [35] and the GWAS Catalog [36] as well as manual review of previously published metabolomics GWAS (Supplementary Methods), suggests 33 of these locus-known metabolite associations are novel. In addition, we identified 401 locus-metabolite associations from the unknown metabolite peak analysis, representing 336 metabolite features, highlighting a large amount of information in the yet-to-be-identified peaks. Fig. 1: Whole Genome Association Study of known and unknown metabolites in the Jackson Heart Study. Flow diagram detailing whole genome association study of the metabolome, main results, and subsequent bioinformatic pipeline for unknown metabolite identification. Rare minor allele frequency is defined as <1% in NFE using gnomAD. Confirmation of metabolite identities was limited to commercially available metabolite standards. WGAS whole genome association study, MS mass spectrometry; NFE non-Finish Europeans, GNPS global natural product social networking. Full size image Fig. 2: Phenogram of 519 locus-metabolite relationships in the Jackson Heart Study. 118 loci-metabolite associations are for known metabolites. 401 associations are for unknown metabolite features. The most common metabolite class includes amino acids, peptides, and analogs. Highlighted are sentinel genes with ≧ 4 locus-metabolite associations. Full size image Of the 226 metabolite quantitative trait loci (mQTLs), there were 159 unique genes annotated as the lead candidate gene (closest protein-coding gene to the mQTL). Of the sentinel SNPs, 65% were expression quantitative loci (eQTL) for their corresponding gene as determined by PhenoScanner v2.0 ( p value <2E-4; Supplementary Data 2 ). Of those that were not eQTLs for the candidate gene, the majority were rare in individuals of non-Finnish European Ancestry (MAF <1% in gnomAD), highlighting a key limitation of presently available genomic information when performing investigations in Black individuals. Among the sentinel SNPs, 22% were located in exons and an additional 19% were in enhancer or promoter regions (Fig. 3 and Supplementary Data 2 ). Fig. 3: Genetic architecture of metabolite-WGAS associations. A Number of metabolites associated with each locus; B Absolute distance from mQTL position to transcription start site; C Minor allele frequency and effect size; D Frequency of mQTL sentinel allele in non-Finnish European Individuals vs African individuals; E Location of mQTL . WGAS whole genome association study, mQTL metabolite quantitative loci. Full size image Of the 519 locus-metabolite associations meeting the Bonferroni level of significance, 368 locus-metabolite peak relationships were available for validation in both MESA and HERITAGE, of which 91% were validated with a p value <0.05 and consistent direction of effect. An additional 100 locus-metabolite peak associations were available in either MESA or HERITAGE, of which 86% were validated. Overall, there was 90% validation of available locus-metabolite associations with p value <0.05; 68% validation (318 of 468 locus-metabolite associations available) using Bonferroni level of significance (0.05/468; p value <1E-4; Supplementary Data 2 ). Ancestry-specific variants and metabolite associations WGS of diverse populations provides an opportunity to assess allelic architectures of populations of different ancestries and inform underlying biology. In particular, for our study, 17% of the 226 sentinel SNPs that were rare (MAF <1%) in Non-Finnish Europeans were common in individuals of African ancestry (MAF >5%; Supplementary Data 2 ). Overall, 29% of the sentinel SNPs were nearly monoallelic in individuals of NFE ancestry with a MAF <0.01% in gnomAD [37] . Here, we highlight several novel locus-metabolite relationships with SNPs that are rare in NFE (Table 1 ). Table 1 Ancestry-specific mQTLs in the Jackson Heart Study Full size table As an example, The TTR variant (V122I) is present in 3–4% of Black individuals and has been implicated in the pathophysiology of heart failure in the elderly, often unrecognized. We found the V122I in TTR to be associated with an unknown metabolite ( m/z 269.226) in JHS (ß = − 0.76, p value = 4.4E-14). The TTR tetramer complexes with retinol-binding protein (RBP4). This metabolite peak is correlated with RBP4 ( r 2 = 0.64) measured by aptamer-based proteomic profiling [38] and V122I is significantly associated with RBP4 levels in JHS. Leveraging MS/MS data and its genetic association with TTR and correlation with RBP4, we predicted this compound to be all- trans -retinol (vitamin A), which we subsequently confirmed with an authentic standard (Supplementary Fig. 1 ). In addition, another variant that is nearly monoallelic in individuals of European ancestry, in APOE (rs769455), is associated with an unknown metabolite peak ( m/z 269.226; ß = 0.71, p value = 1.5E-12) that has an identical molecular mass to all -trans -retinol (Fig. 4 ) and MS fragmentation analysis and MS comparison against chemical standards and all- trans -retinol and other retinol species predicts that it is a cis -isomer of retinol. Fig. 4: Ancestry-specific alleles reveal novel associations of TTR and APOE with retinol species. A Association of V122I in TTR with an unknown metabolite (QI722; m/z 269.226 ); B Correlation between QI722 and retinol-binding protein; C Association of rs769455 missense variant in APOE with unknown metabolite (QI176; m/z 269.226); D TTR associated unknown metabolite matching spectra with trans-retinol; APOE associated unknown metabolite with identical molecular mass but earlier retention time indicating it’s a cis -isomer of retinol. Additional isomers tested without compound match include 9 and 11- cis retinol. Full size image Annotation for unknown metabolite peaks associated with genomic loci Of the 2291 metabolites measured, 1954 were unknown metabolite peaks, of which 336 were associated with genomic loci ( p value <8E-11). Of the mQTLs associated with unknown features, 15 had no prior metabolite associations within 500 kb of the sentinel SNP; 12 of these SNPs were rare in individuals of NFE ancestry. (Supplementary Data 2 ). In the first step of assigning chemical identities to unknown metabolites, we clustered metabolite peaks measured in the positive mode (known and unknown metabolites) to identify primary metabolite features and their adducts (Supplementary Data 3 ). After applying our clustering algorithm, 49 of the 336 unknown metabolite peaks were part of clusters with known metabolites and were assigned the chemical identity of this primary metabolite. Of the 287 unknown metabolites not clustered with known compounds, 63 were adducts or fragments of other primary unknown metabolites, leaving 224 as major ions or primary unknown metabolites (Fig. 5 ). Fig. 5: Unknown metabolite annotation pipeline using bioinformatic tools leveraging MS/MS spectra. Unknown metabolite identification with initial clustering of features to elucidate adducts and fragments of primary features or major ions. Subsequent implementation of tools leveraging MS/MS data, including SIRIUS, GNPS, and CANOPUS. Metabolite ID validation is limited to commercially available standards. Full size image Next, to aid in the identification of the unknown metabolites, we applied MS/MS profiling to metabolite peaks measured in positive mode, resulting in MS/MS data on 91% of unknown metabolite peaks designated as major ions or primary metabolites in our study. Using CANOPUS [39] , a bioinformatics tool which uses MS/MS data to annotate chemical compound class for metabolites, 72% of primary unknown metabolite features were assigned a metabolite compound class; lipids, amino acids, and fatty acids were the most common metabolite groups. SIRIUS [40] , a software tool that uses MS/MS data for metabolite structural elucidation, assigned chemical predictions in rank order for 182 primary unknown metabolites received (top three metabolite predictions for each feature in Supplementary Data 3 ). Leveraging these chemical predictions, we assigned high-confidence metabolite IDs to 33 metabolites that carried additional evidence for supporting the annotation using complementary tools, including Global Natural Product Social Molecular Networking (GNPS; n = 8) [41] , a database for MS/MS spectra in metabolomics studies, and the Human Metabolome Database (HMDB; n = 5) [32] , MS data for related compounds from our in-house metabolite library ( n = 12) or validation with chemical standards ( n = 8). In addition to providing a database of MS/MS data for metabolomics studies, GNPS allows visualization of networks of structurally similar metabolites based on MS fragmentation data within studies to derive metabolite identities. As an example, chemical annotation using SIRIUS failed to generate a high-confidence metabolite prediction for an unknown metabolite with m/z 536.4354. However, using GNPS and comparing MS fragmentation data of this metabolite peak to community-based MS/MS spectra repositories, we were able to annotate this peak as carotene. Carotene is associated with rs2293440 (ß = 0.20, p value = 4.73E-11, an exonic variant in Scavenger Receptor Class B Receptor 1 (SCARB1) . SCARB1 plays a key role in lipoprotein metabolism through its action on reverse cholesterol transport and is associated with cholesterol levels in large population genomic studies [42] . Additionally, SCARB1 has been associated with the cellular uptake of carotenoids [43] , increasing our confidence in our metabolite annotation. Using GNPS, we mapped structurally similar unknown metabolites based on MS/MS spectra (Fig. 6A ). A closely related metabolite peak ( m/z 568.427 ) with a cosine similarity score for fragmentation spectra of 0.88 (Fig. 6B ; high similarity score designated as >0.7) was noted to be associated with the Beta-carotene 15,15-dioxegynase (BCO1) and Intestine Specific Homeobox (ISX) loci. BCO1 converts carotenoids to retinal and ISX participates in carotenoid metabolism by regulating the expression of BCO1 [44] . Anchoring our potential metabolite identification on these genomic associations, we searched through related carotenoid species based on mass differences between this peak and carotene and annotated this compound to be a carotenoid, zeaxanthin (Fig. 6D ), which we subsequently validated with a chemical standard. In addition, the GNPS network identified another closely related compound in this network of unknown peaks, cryptoxanthin, a naturally occurring carotenoid compound. Fig. 6: GNPS molecular network identifies carotenoid metabolites linked with genomic loci. A Molecular network of unknown features matching beta-carotene ( m/z 536.4354; identified using MS/MS database) and carotene-related compounds using the Global Natural Products Social Molecular Networking. Nodes represent MS/MS spectra obtained at either discreet collision energies ranging from 10 to 50 V or stepped (SV) collision energies. The circular node shape illustrates whether features are representative ions (highest mean abundance) in clusters of co-eluting features with abundances correlating with Spearman coefficients >0.80. Conversely, square nodes correspond to features that based on correlation with co-eluting compounds, are potentially redundant fragments or adducts. Edges represent the cosine similarity among MS/MS spectra and formulas. Zeaxanthin is the predicted metabolite at m/z 568.427 based on m/z differences and association with BCO1 , which catalyzes the conversion of carotenoids to retinal and ISX , which regulates the expression of BCO1 . B Spectral comparison of plasma unknowns matching carotene and zeaxanthin MS/MS obtained using stepped and discrete collision energy, respectively, illustrating an edge cosine similarity score of 0.88. C Validation of compound identities for zeaxanthin and carotene confirming the retention time match of authentic standards with the unknown features in plasma ( D ) as well as their MS/MS spectrum match. Full size image Of the 37 high-confidence metabolite IDs from unique primary unknown metabolites (33 from SIRIUS predictions with supporting sources of information and four using GNPS; Supplementary Data 6 ), 92% (34/37) were evaluated as having genomic evidence in support of the chemical compound predictions based on the known metabolic pathways of the assigned lead candidate gene (Supplementary Data 2 ). In addition, CANOPUS annotated 29 of the 37 with metabolite class, of which 27 were in support of the metabolite annotation. We confirmed 11 unknown metabolite compound annotations with commercially available chemical standards; five of these are part of novel associations in a metabolomics GWAS: all- trans -retinol, zeaxanthin, 5,6 dihydrouridine, AICA-Riboside, and cholestanone (Supplementary Data 3 and Supplementary Fig. 1 ). MS/MS data on all metabolites associated with genomic loci in our study are made available (Supplementary Data 7 ). In the present study, we used WGAS to identify genetic determinants of plasma metabolites in a Black population from JHS and applied novel chemical profiling and bioinformatic methods to annotate unknown metabolite peaks. In our cohort of Black individuals, the presence of ancestry-specific alleles that are nearly monoallelic in individuals of European ancestry increases the power to detect novel metabolomic associations with established cardiovascular risk loci—and represents an important first step in the broader discovery of ancestry-specific, pathogenically significant metabolic differences. In this study, we show a novel association in a clinically relevant polymorphism in TTR (Transthyretein) , which is associated with increased risk of heart failure in Black individuals, and an unknown metabolite feature we identify as all- trans- retinol. The TTR V122I polymorphism described in 3–4% of Black individuals destabilizes the TTR-RBP4 tetramer, thereby displacing RBP4 and promoting amyloid fibril formation that precipitates heart failure and death [45] . The reduced circulating all-trans retinol observed in our study may similarly be related to increased clearance and a potential marker of TTR-RBP4 tetramer stability, as has been postulated in cases with ATTRv V122I amyloidosis [45] . The effect of reduced all-trans retinol on downstream active retinol metabolites, including retinoic acid, and its potential contribution toward pathologic cardiac hypertrophy needs further study. The Apolipoprotein E locus is a complex genomic region encoding APOE and the isoforms produced from its polymorphic alleles. APOE is involved in critical metabolic pathways, including lipid transport and metabolism [46] , and is associated with chronic diseases, including the development of atherosclerosis and Alzheimer’s disease, presumably mediated by its role in the transport and clearance of cholesterol and amyloid peptides to the brain [47] . We show an association between a missense variant in APOE (rs769455), a nearly monoallelic polymorphism in individuals of European ancestry, with an unknown metabolite peak ( m/z 269.226). This unknown metabolite has an identical molecular mass to all -trans -retinol and MS fragmentation analysis suggests that it is a potential isomer of retinol. While retinyl esters form with chylomicrons transported by APOE, the role of APOE transport on retinol species and potential downstream implications for retinoid transport and bioavailability has yet-to-be elucidated. Variants near retinoic acid transporters and receptors (downstream and active metabolites of retinol) have shown associations with risk for Alzheimer’s disease and defective transport of retinol and related species has been implicated in this disease [48] , [49] . Our findings showing associations between APOE and cis -retinol may have potential implications for the biological roles of APOE in disease pathways. We show a novel association between an ancestry-specific variant in CD36 ( Platelet Glycoprotein IV; rs3211938) associated with specific plasmalogens, a subclass of phospholipids integral to cell membrane signaling and stability. CD36 is an integral transmembrane protein involved in the sequestration of malarial species, plasmodium falciparum , preventing splenic destruction of the organisms. As such, variants in CD36 offer protection against malaria infection [50] . In addition, CD36 functions as a receptor for several important inflammatory mediators, fatty acids, and lipids among others, and is implicated in processes including regulation of blood pressure [51] , lipids [52] , and the development of atherosclerosis in model systems [53] , [54] , [55] . Novel associations of CD36 with plasmalogen species, which are glycerophospholipids with important antioxidant properties and have been associated with the protection of endothelial cells in hypoxic conditions [56] , as well as with cell signaling and membrane stability [50] , highlight potential lipid mediators, and mechanisms for the role of CD36 in cardiometabolic disease development. Sickle cell anemia is characterized by severe vascular abnormalities and leads to chronic cardiovascular diseases, including pulmonary hypertension, heart failure, and stroke [57] . In addition, individuals with the sickle cell trait are also at increased risk of developing chronic kidney disease [58] . Our findings show an association between the sickle mutation, rs334 , and an unknown metabolite which we predict to be a lysophosphatidylcholine, a major component of red blood cell membranes. Red blood cell membrane structure is significantly altered in individuals with sickle cell disease, which affects cell shape, hemodynamics, and protein-membrane signaling interactions [59] . This metabolite association may be a marker of red blood cell membrane remodeling that occurs in sickle cell disease and may help elucidate mechanisms of red blood cell pathology and resulting downstream complications of ischemic and inflammatory tissue damage. Unknown metabolomic profiling presents an opportunity for unbiased discovery in metabolomics GWAS. However, given the breadth and diversity of the metabolome, annotating metabolite peaks with subsequent validation of proposed metabolite identities is a lengthy and arduous process, traditionally requiring extensive manual curation of study features against reference databases. To facilitate a more efficient annotation pipeline for large-scale metabolomics GWAS, we performed additional tandem MS profiling to obtain MS fragmentation data for all our peaks and implemented recently developed bioinformatic methods that leverage MS/MS spectra in metabolomics studies to help annotate unknown compounds with chemical and/or class identities. Individual methods can help elucidate chemical identity by detailing compound sub-structure (SIRIUS), structural similarity to other metabolomic features (GNPS), and compound class (CANOPUS). In our study, no one method provided a complete annotation of study features, highlighting the challenges and complexity of working with unknown metabolomics. However, the use of complementary tools to elucidate metabolite identities enabled structural and/or class annotation for a majority of profiled peaks and represents the first systematic application of these bioinformatic tools to identify unknown peaks in a genomic association study. We have previously demonstrated how genomic integration with MS fragmentation data on unknown metabolite peaks can help narrow the focus for these features, by mapping loci to predicted compounds based on shared metabolic pathways [34] . Here we have systematically integrated genetic associations with MS/MS spectra-based metabolite predictions from bioinformatic techniques. We find that a majority of our metabolite annotations, based on chemical identity, can be mapped to the metabolic/functional pathway of the associated lead candidate gene, providing an additional layer of support as we decipher metabolite identities associated with cardiometabolic diseases. As an example, an unknown metabolite feature with m/z 259.1036 is associated with triglycerides, DM, and CHD among other traits in JHS (Supplementary Data 4 ). This metabolite peak maps to the ATIC gene, which encodes 5-Aminoimidazole-4-Carboxamide Ribonucleotide Formyl transferase/IMP Cyclohydrolase , a protein-coding gene involved in purine biosynthesis. One of the top computational predictions based on tandem MS for this metabolite was AICA-Riboside (Acedesine). While this compound has been described as an AMP-activated protein kinase agonist with investigational applications in treatments for diabetes and lymphoma [60] , [61] , [62] , there is evidence that endogenous levels of the compound are physiologically important. ATIC deficiency, a recessive genetic disease, results in impaired purine synthesis and increased urinary AICA-Riboside and is marked by severe neurodevelopmental delays, growth impairment, and dysmorphic features [63] , [64] . The association of AICA-Riboside, with its canonical enzymatic pathway in WGAS, narrowed our metabolite search to this single bioinformatic prediction, which we then confirmed with a commercial standard (Supplementary Fig. 1 ). Thus, the integration of genetics and MS/MS spectra can sometimes enable an efficient pipeline for identification of metabolites associated with cardiometabolic disease. Our study represents one of the few analyses of genome-metabolome integration in a Black population. As such, validation of locus-metabolite associations presents a significant challenge, especially for associations in ancestry-specific alleles, given the scarcity of both known and unknown metabolomics profiling in Black populations. In addition, metabolomics GWAS have traditionally implemented genotype imputation of SNP array using reference panels. However, in an admixed population such as JHS, limited representative reference panels necessitate the use of more accurate imputation panels or whole genome sequencing. Further efforts to apply metabolomic profiling in Black populations and integrate with WGS will be essential to replicate key locus-metabolomic findings, though many have strong biologic plausibility. To assess the novelty of our findings, we used the most up-to-date genomic databases assessing genotype-phenotype associations, as well as a manual review of prior published metabolomics GWAS. However, there is the potential that we may have missed some previously published locus-metabolite associations. In addition, though we have made significant progress in compound identification for unknown metabolite features, a significant number still lack validation with chemical standards, and there may be some inaccuracies in chemical and/or compound class annotations, though we believe the integration of genetic findings and novel bioinformatic tools have helped minimize misclassification. While we will continue to systematically validate these compound IDs, we make available our sample library of MS/MS spectra with clinical and genomic associations, which can be leveraged across the omics community, providing a crowdsourcing opportunity for metabolite identification and serving as an ongoing resource for validation of metabolite peaks. In summary, our integrative approach toward the identification of known and unknown metabolites involved in diverse disease processes using WGAS in a Black population highlights novel and clinically relevant locus-metabolite associations. In addition, genomic integration with advanced chemical phenotyping using tandem MS improves the ability to annotate unknown metabolite peaks, the “dark matter” of the metabolome. This sample library of MS/MS spectra of metabolite features linked to genomic loci and clinical traits will improve the identification of biologically relevant metabolites. Cohorts The study designs and methods for JHS, MESA, and HERITAGE have been described in refs. 65 , 66 , 67 . JHS is a prospective population-based observational study designed to investigate risk factors for cardiovascular disease (CVD) in Black individuals. In 2000–2004, 5306 Black individuals from the Jackson, Mississippi tri-county area (Hinds, Rankin, and Madison counties) were recruited for a baseline examination. Of the original cohort, 2466 individuals had whole genome sequencing and metabolomic profiling performed from baseline fasting samples and were included in the analyses. MESA included 6814 participants between the ages of 45–84 years recruited at six clinical centers across the US, who were identified as members of four racial/ethnic groups: White, Hispanic, Asian, or Black (28%). Included in the present study are 995 individuals across all four racial/ethnic groups with metabolomic profiling and WGS at baseline exam. HERITAGE enrolled a combination of self-identified white and Black family units, totaling 763 sedentary participants (38% Black) between the ages of 17–65 years, in a 20-week, graded endurance exercise training study across four clinical centers in the US and Canada in 1995. Included in the present study is a random subset of 658 individuals with baseline metabolomic profiling and genotyping. Study approval The Institutional Review Boards of Beth Israel Deaconess Medical Center, University of Mississippi Medical Center, University of Washington (MESA), and HERITAGE clinical centers approved the human study protocols, and all participants provided written informed consent. LC-MS metabolite profiling Metabolite profiling was performed using two LC-MS methods. Organic acids and other intermediary metabolites were separated using amide chromatography (Waters XBridge Amide column) and measured using targeted negative ion mode multiple reaction monitoring (MRM) MS with an LC-MS system comprised of an Agilent 1290 infinity LC coupled to an Agilent 6490 triple quadrupole mass spectrometer. MRM data were processed using Agilent Masshunter QQQ Quantitative analysis software [68] . Separately, amino acids, acylcarnitines, and other polar metabolites (including both known and unknown metabolite features) were separated using hydrophilic interaction liquid chromatography (HILIC) using an Atlantis HILIC column (Waters; Mildford, MA) and measured using nontargeted, full scan, high-resolution MS in the positive ion mode over m/z 70–800 with an LC-MS system comprised of a Nexera X2 U-HPLC (Shimadzu Corp.; Marlborough, MA) coupled to a Q Exactive mass spectrometer (Thermo Fisher Scientific; Waltham, MA). Raw data were processed using TraceFinder 3.3 (Thermo Fisher Scientific; Waltham, MA) for supervised integration of a subset of identified metabolites and quality control. Progenesis QI (Nonlinear Dynamics; Newcastle upon Tyne, UK) was used for the detection and integration of both identified and unknown features. Each feature in the dataset was tracked by its measured mass to charge ratio and chromatographic retention time, which serves as a unique “tag” for each LC-MS peak. Known compounds were annotated using mixtures of authentic reference standards analyzed with each batch and reference data. These metabolites had previously been annotated in human plasma and confirmed via spiking experiments with standards and by matching retention times and MS data. Metabolites with a coefficient of variation [69] greater than 30% and those missing in more than 30% of measured samples were removed from the analysis [70] . Isotope-labeled internal standards were monitored in each sample to ensure proper MS sensitivity for quality control. Pooled plasma samples were interspersed at intervals of 20 participant samples in the HILIC method and intervals of 10 participant samples in the amide chromatography method to enable correction of drift in instrument sensitivity over time and to scale data between batches. We used a linear scaling approach to the nearest pooled plasma sample in the queue. An additional pooled plasma sample was interspersed at every 20 injections to determine the coefficient of variation for each metabolite and unknown over the run. Peaks were manually reviewed in a blinded fashion to assess quality. MS/MS data acquisition We acquired product ion mass spectra (MS/MS) on unknown features to aid their identification. All MS/MS data were acquired using an LC-MS system comprised of a Nexera X2 U-HPLC (Shimadzu Corp.; Marlborough, MA) coupled to an ID-X orbitrap mass spectrometer (Thermo Fisher Scientific; Waltham, MA). LC conditions were identical to those used in the nontargeted HILIC method, and electrospray ionization MS settings were spray voltage 3.5 kV, sheath gas 40, sweep gas 2, capillary temperature 350 °C, heater temperature 300 °C, S-lens RF 40. MS/MS data were generated using a combination of data-dependent acquisition (DDA) and inclusion list-directed MS/MS acquisition. For DDA, we used the AcquireX pipeline provided with the Thermo ID-X instrument and five consecutive injections of the JHS pooled plasma sample used for QC. The AcquireX scan cycle included an MS survey scan (70–800 m/z) followed by five MS/MS scans with a stepped collision energy of 10, 25, and 50 eV. To obtain MS/MS data on features not captured by the unsupervised AcquireX approach, we also used a directed MS/MS data acquisition approach in which lists of specific ions and retention time windows (inclusion lists) were created as required to measure spectra for ions of interest. First, we split all features in the study into 24 individual mass inclusion lists, separated based on ranges of metabolite peak retention times obtained from the initial LC-MS experiment, to improve the sensitivity of MS/MS data acquisition. We then generated MS/MS spectra using higher-energy C-trap dissociation (HCD) with stepped collision energies (10, 25, 50 V). Second, we targeted unknown features with GWAS hits and generated MS/MS with an expanded set of collision energies ranging from 10 to 50 V in 10 V increments. In order to increase the likelihood of capturing low abundance features in the JHS pool pooled plasma, samples used for MS/MS acquisition were concentrated ten-fold. Metabolites were extracted from 100 µL of pooled plasma using 900 µL of 74.9:24.9:0.2 (v/v/v) acetonitrile/methanol/formic acid. The samples were centrifuged (10 min, 9000× g , 4 °C) and the supernatants were dried under a gentle stream of nitrogen gas TurboVap LV, Biotage). Dried extracts were resuspended in 100 µL of 10:67.4:22.4:0.18 (v/v/v/v) water/acetonitrile/methanol/formic acid containing stable isotope-labeled internal standards (valine-d8, Sigma-Aldrich; St. Louis, MO; and phenylalanine-d8, Cambridge Isotope Laboratories; Andover, MA) and 10 µL were injected per LC-MS/MS analysis. MS/MS data processing Raw files were converted to *.mzML format files using MSConvert [71] and both extracted ion chromatograms [37] and matching MS/MS scans for each individual feature were generated using the R package MSnbase v. 3.12 [72] , and in-house scripts for producing EIC and MS/MS spectra visualizations. Feature retention times and peak quality in the concentrated pools were confirmed by visually inspecting the chromatography peak shapes of each individual feature. After confirming the study retention times in the MS/MS acquisition, the extraction of MS/MS data was conducted by finding scans with precursors within ±0.2 a.m.u. of the known features and ±0.1 min from the apex of the peak detected in the MS/MS run. Matching MS/MS peaks within 5 ppm across MS/MS scans spanning the range were aggregated whenever more than one MS/MS scan was mapped to each individual feature. The resulting peak height for aggregated peaks was determined as the average of the aggregated peak intensities. Peaks inconsistently detected across MS/MS scans were removed from the final MS/MS inventory. Additionally, an electronic noise fragment detected in the MS/MS of low abundance peaks within 30 ppm of m/z of 173.46 was removed from parsed data. Parsed MS/MS was formatted as input for molecular structure predictions (*.ms) or MS/MS-based similarity networks (*.MGF). For MS/MS-based similarity predictions, spectra generated for individual features using more than one collision energy were kept as independent molecular features. Genotyping Whole genome sequencing (WGS) in JHS and MESA has been described in ref. 73 . Participant samples underwent >30× WGS through the Trans-Omics for Precision Medicine project at the Northwest Genome Center at the University of Washington and the Broad Institute and joint genotype calling with participants in Freeze 6; genotype calling was performed by the Informatics Resource Center at the University of Michigan. Genotyping in HERITAGE was performed on the Illumina Infinium Global Screening Array. Genotypes were called using Illumina’s GenCall based on the TOP/BOT strand method. Genotype imputation to the TOPMed Freeze5 reference panel was performed using the University of Michigan Imputation Server Minimac4. In addition, phasing was performed with Eagle v2.4. Sites with call rates <90%, mismatched alleles, or invalid alleles were excluded. Whole genome association study Metabolite LC-MS peak areas were log-transformed and scaled to a mean of zero and standard deviation of 1 and subsequently residualized on age, sex, batch, and principal components (PCs) of ancestry 1–10 as determined by the GENetic EStimation and Inference in Structured samples (GENESIS) [74] , and subsequently inverse normalized. The association between these values and genetic variants was tested using linear mixed-effects models adjusted for age, sex, the genetic relationship matrix, and PCs 1–10 using the fastGWA model implemented in the GCTA software package [75] . Variants with a minor allele count less than 5 in a given cohort were excluded from analysis in that cohort. A Bonferroni adjusted significance threshold of 8E-11 (5 × 10 −8 /602 PC’s explaining 95% of the variance of metabolite levels) was used for discovery in JHS. To identify sentinel SNPs and metabolite quantitative loci (mQTL), we first defined a 1 Mb region around each SNP significantly associated with a given metabolite. Starting at the SNP with the lowest p value, overlapping mQTLs for a particular metabolite were merged. This process was repeated until no more overlapping regions existed for the given metabolite, and the lead variant was identified as the one with the lowest p value. Lead variants that were not in overlapping regions but in linkage disequilibrium (LD) with r 2 ≥ 0.8 were again combined using SNPClip [76] , and this final merged region was designated as the mQTL, with the most significant SNP retained as the sentinel variant. Where association statistics were available in both MESA and HERITAGE, the two cohorts were meta-analyzed by the inverse-variance weighted method using the “metagen” package in R. Validation threshold was set at p < 0.05 with a consistent direction of effect. Variant annotations Reference allele frequencies from gnomAD and variant functional annotations using GENCODE and ClinVar disease annotations were obtained from the Functional Annotation of Variants—Online Resource (available favor.genohub.org, download date August 1, 2020). Comparing to previous mQTLs We used existing genomic databases and prior blood metabolomics GWAS to assess the novelty of our locus-metabolite associations. To determine whether mQTLs of known metabolites were novel, we first utilized the PhenoScanner package for R. A 1 MB region around each sentinel SNP associated with a metabolite was passed to the PhenoScanner function in R: build was set to “38”, p value to 5 × 10 −8 , catalog to “mQTL” (query date 12/1/2021). Novel locus-metabolite associations were cross-referenced against the GWAS Catalogue using the sentinel SNP and a 1 MB surrounding region. In addition, gene-metabolite associations were manually reviewed for novelty across 21 published GWAS of metabolomics (details of individual studies reviewed in Supplementary Methods) [3] , [4] , [5] , [6] , [7] , [8] , [9] , [10] , [11] , [12] , [13] , [14] , [15] , [16] , [17] , [18] , [19] , [20] , [21] , [22] , [23] . mQTL and phenotype associations To determine overlap between clinical GWAS analyses and mQTLs in this analysis, we utilized the PhenoScanner package for R. All sentinel SNPs associated with metabolite peaks as identified above were passed to the PhenoScanner function in R with the following arguments: build was set to “38”, p value to “1 × 10 −5 ”, catalog to “GWAS”, r2 was set to “0.8”, proxies set to “None” (query date 12/1/2021). Unknown metabolite peak annotation Metabolite peak clustering The electrospray ionization process used in LC-MS can generate more than one type of ion adduct of a molecule (e.g., [M + H] + , [M + Na] + , etc. ), partially fragment molecules, and generate multimer ions. A single metabolite may therefore give rise to multiple unknown peaks. However, such redundant features share the same chromatographic retention time and have highly correlated signal intensities. To filter redundant features, all profiled metabolite peaks (HILIC platform) were grouped into clusters based on a retention time similarity of ±0.25 min and a signal intensity spearman correlation coefficient >0.80. The [M + H] + ion, if identified by mass differences among features in the cluster or the feature with the highest signal intensity, was identified as the primary feature. Metabolite annotations leveraging MS/MS spectra and bioinformatic tools Parsed MS/MS data (*.ms) were loaded into SIRIUS CSI-Finger ID version 4.7.2 [40] . Molecular formula predictions generated with Orbitrap-specific settings (MS/MS isotope scorer: ignore, mass deviation: 5 ppm, Candidates: 10, Candidates per ion: 1, possible ionizations: [M + H] + , [M + K] + , [M + Na]+). Structure elucidations were done using PubChem and the adducts [M + H] + , [M + K] + , [M + Na]+). Predictions were exported and the top three structure elucidations were parsed for each feature. Parsed MS/MS data for each metabolite peak were annotated for predicted metabolite class using ClassyFire ontology through CANOPUS [39] . MS/MS-based networks were built using the Global Natural Products Social Molecular Networking (GNPS) [41] , and the resulting networks were visualized with Cytoscape v. 3.8.2 [77] . To provide supporting information for our metabolite annotations, we searched the Human Metabolome database with m/z ± 5 ppm [32] . Metabolite annotation scheme Results from metabolite feature clustering, class, and chemical structure elucidations were integrated to annotate metabolite peaks. We subsequently assigned each annotation to a category based on levels of supporting evidence. 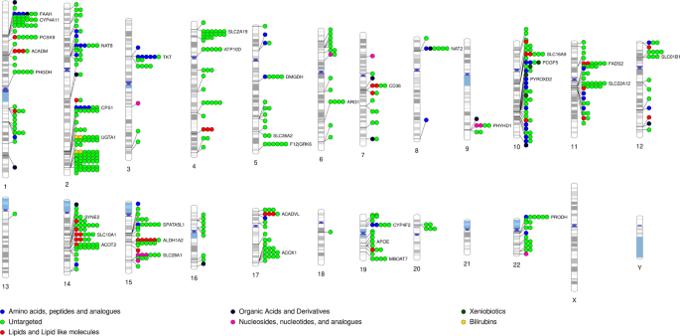Fig. 2: Phenogram of 519 locus-metabolite relationships in the Jackson Heart Study. 118 loci-metabolite associations are for known metabolites. 401 associations are for unknown metabolite features. The most common metabolite class includes amino acids, peptides, and analogs. Highlighted are sentinel genes with≧4 locus-metabolite associations. In addition, we classified the categories of metabolite identification in accordance with the Metabolomics Standards Initiative (MSI) recommendations (Supplementary Table 2 ): [78] Category 1: metabolite match to an authentic reference standard; Category 2: metabolite clusters with a known compound which has previously validated with standard (Category 1 and 2 corresponds to MSI Classification 1 as Identified Metabolite); Category 3: metabolite with MS/MS-based GNPS database match (MSI Classification 2: putatively annotated metabolite); Category 4: Metabolite with similar MS/MS spectra and retention time with the representative backbone of chemical standard for a compound in the metabolite family (manual curation) using in-house metabolite library (MSI classification 3: putatively annotated metabolite class). In addition, we add category 5: SIRIUS MS/MS-based chemical formula/compound predictions and Category 6: compound match using m/z search in HMDB, which are not included in the 2007 MSI classification scheme. Primary unknown metabolites with multiple sources of supporting evidence represented high-confidence metabolite annotations and were assigned specific metabolite IDs. Genomic and metabolite pathway integration Genetic associations with unknown metabolite peaks can be integrated with MS/MS and bioinformatic metabolite annotations in an effort to further illuminate metabolite identifications and/or offer supporting evidence for predictions based on the known pathways of the locus. 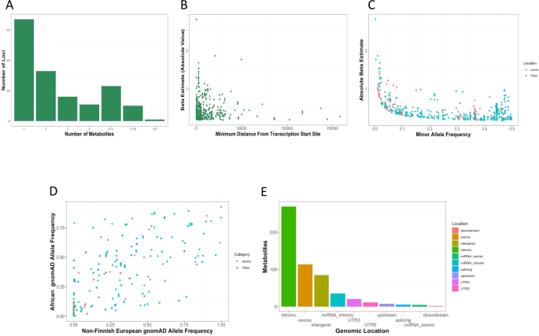Fig. 3: Genetic architecture of metabolite-WGAS associations. ANumber of metabolites associated with each locus;BAbsolute distance from mQTL position to transcription start site;CMinor allele frequency and effect size;DFrequency of mQTL sentinel allele in non-Finnish European Individuals vs African individuals;ELocation of mQTL.WGAS whole genome association study, mQTL metabolite quantitative loci. Each lead candidate gene (nearest gene to sentinel SNP) was annotated for its associated metabolic pathways using the KEGG database [79] . 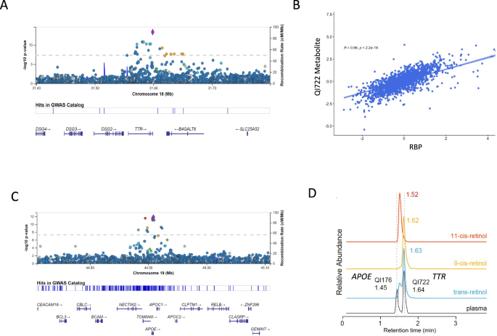Fig. 4: Ancestry-specific alleles reveal novel associations of TTR and APOE with retinol species. AAssociation of V122I inTTRwith an unknown metabolite (QI722;m/z 269.226);BCorrelation between QI722 and retinol-binding protein;CAssociation of rs769455 missense variant inAPOEwith unknown metabolite (QI176; m/z 269.226);DTTRassociated unknown metabolite matching spectra with trans-retinol;APOEassociated unknown metabolite with identical molecular mass but earlier retention time indicating it’s acis-isomer of retinol. Additional isomers tested without compound match include 9 and 11-cisretinol. Metabolite annotations were evaluated in the context of the metabolic pathways of the candidate gene or its prior GWAS associations to assess whether there was genomic evidence in support of the chemical compound identification. 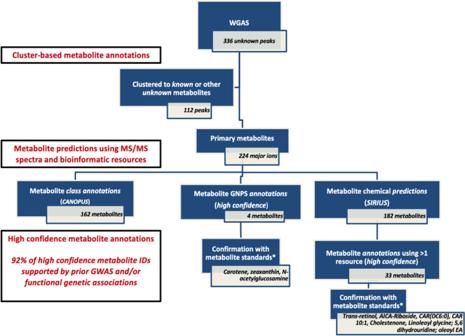Fig. 5: Unknown metabolite annotation pipeline using bioinformatic tools leveraging MS/MS spectra. Unknown metabolite identification with initial clustering of features to elucidate adducts and fragments of primary features or major ions. Subsequent implementation of tools leveraging MS/MS data, including SIRIUS, GNPS, and CANOPUS. Metabolite ID validation is limited to commercially available standards. 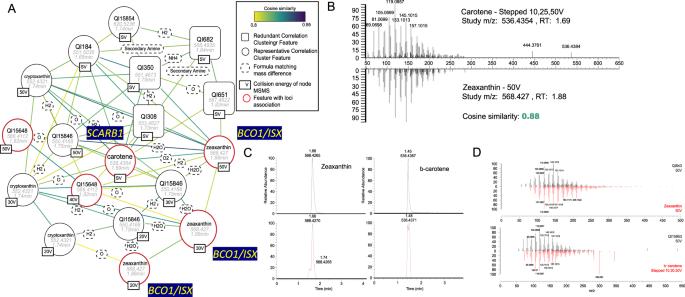Fig. 6: GNPS molecular network identifies carotenoid metabolites linked with genomic loci. AMolecular network of unknown features matching beta-carotene (m/z536.4354; identified using MS/MS database) and carotene-related compounds using the Global Natural Products Social Molecular Networking. Nodes represent MS/MS spectra obtained at either discreet collision energies ranging from 10 to 50 V or stepped (SV) collision energies. The circular node shape illustrates whether features are representative ions (highest mean abundance) in clusters of co-eluting features with abundances correlating with Spearman coefficients >0.80. Conversely, square nodes correspond to features that based on correlation with co-eluting compounds, are potentially redundant fragments or adducts. Edges represent the cosine similarity among MS/MS spectra and formulas. Zeaxanthin is the predicted metabolite atm/z568.427 based onm/zdifferences and association withBCO1, which catalyzes the conversion of carotenoids to retinal andISX, which regulates the expression ofBCO1.BSpectral comparison of plasma unknowns matching carotene and zeaxanthin MS/MS obtained using stepped and discrete collision energy, respectively, illustrating an edge cosine similarity score of 0.88.CValidation of compound identities for zeaxanthin and carotene confirming the retention time match of authentic standards with the unknown features in plasma (D) as well as their MS/MS spectrum match. Reporting summary Further information on research design is available in the Nature Research Reporting Summary linked to this article.